Decreased tumorigenesis in mice with aKraspoint mutation at C118 KRAS, NRAS or HRAS genes are mutated to encode an active oncogenic protein in a quarter of human cancers. Redox-dependent reactions can also lead to Ras activation in a manner dependent upon the thiol residue of cysteine 118 (C118). Here, to investigate the effect of mutating this residue on tumorigenesis, we introduce a C118S mutation into the endogenous murine Kras allele and expose the resultant mice to the carcinogen urethane, which induces Kras mutation-positive lung tumours. We report that Kras +/ C118S and Kras C118S / C118S mice develop fewer lung tumours. Although the Kras C118S allele does not appear to affect tumorigenesis when the remaining Kras allele is conditionally oncogenic, there is a moderate imbalance of oncogenic mutations favouring the native Kras allele in tumours from Kras +/ C118S mice treated with urethane. We conclude that the Kras C118S allele impedes urethane-induced lung tumorigenesis. The Ras family of small GTPases, comprised of the KRAS , NRAS and HRAS genes, are mutated to encode constitutively active, GTP-bound, oncogenic proteins in upwards of one quarter of all human cancers, which is well established to promote tumorigenesis [1] . Despite the prominent role these genes play in human cancer, the encoded proteins have proven difficult to pharmacologically inhibit [2] , [3] . As such, it is important to understand how Ras proteins are activated. In this regard, Ras proteins cycle between GDP-bound inactive and GTP-bound active states, the latter being catalysed by guanine nucleotide exchange factors (GEFs) [4] , [5] . GEFs are not, however, the only means of activating Ras proteins. Free radical oxidants can lead to S -nitrosylation or S -glutathiolation and activation of Ras in a manner dependent on the thiol residue of cysteine 118 (C118) [6] , [7] , [8] . Accumulating evidence supports the possibility that such redox-dependent reactions with C118 may have cellular consequences. Specifically, an increase in S -nitrosylation and activation of Ras can stimulate MAP-kinase (MAPK) signalling [6] , [9] , [10] , [11] , [12] , [13] , [14] , phosphatidylinositol 3-kinase signalling [15] and/or cell proliferation [16] . Similarly, an increase in S -glutathiolation and activation of Ras impacts a variety of signalling pathways in a manner apparently dependent upon C118 (refs 17 , 18 ). Finally, reducing the expression of endothelial nitric oxide synthase (eNOS), which catalyses the production of nitric oxide [19] , decreases the levels of S -nitrosylated and active Ras as well as xenograft tumour growth in a number of cancer cell lines [20] . Despite accumulating data, the effect of specifically blocking redox-dependent reactions with C118 on the function of endogenous mammalian Ras remains to be explored in vivo. This is especially important in terms of cancer, as tumour initiation appears to be sensitive to the level of activated Ras [21] . Fortunately, there is a very precise separation-of-function mutation that apportions these effects from other functions of Ras. Specifically, substitution of C118 for serine (C118S), a very minor modification in which the thiol residue of this cysteine is replaced with a hydroxyl group, renders Ras completely insensitive to activation by free radical-mediated oxidants, with no measureable effect on the protein structure, GTPase activity, intrinsic and GEF-mediated guanine nucleotide dissociation rate, or the ability to bind an effector [6] , [8] , [10] , [12] , [17] , [18] , [22] , [23] , [24] . Thus, here we assess the consequences of introducing the C118S mutation into the endogenous murine Kras gene on tumorigenesis in vivo , and find a reduction in carcinogen-induced lung tumorigenesis in mice bearing this mutated allele. Generation of mice with a Kras C118S allele To investigate the effect of mutating C118 on Ras function in vivo during tumorigenesis, a targeting vector was created to insert a single-point mutation, namely a G353 transversion to C (G353>C) encoding the C118S mutation, into exon 3 of the murine Kras gene ( Fig. 1a ). C118S was chosen because this precise separation-of-function mutation specifically blocks the redox-dependent reactions at this site that lead to Ras activation [6] , [8] , [10] , [12] , [17] , [18] , [22] , [23] , [24] . Kras was chosen, as this is the isoform most commonly mutated in human cancers [1] . This vector was electroporated into embryo stem (ES) cells, and cells were selected for resistance to G418 and ganciclovir. Successful recombination events in resistant clones were verified by reverse transcription (RT)–PCR and sequencing to contain the G353>C transversion in Kras ( Fig. 1b ). One such clone was used to generate a founder Kras +/C118S(Neo) mouse, the genotype of which was identified by PCR amplification from genomic DNA. A 314-bp product unique to the targeted Kras C118S(Neo) allele was amplified ( Supplementary Fig. 1a ) using primers anchored in exon 3 of the Kras gene and in the Neo gene of the targeting vector (P3 and P4, Fig. 1a and Supplementary Table 4 ), whereas a 621-bp product unique to the wild-type Kras allele was amplified ( Supplementary Fig. 1a ) using primers anchored in exon 3 and in the adjacent intron (P3 and P5, Fig. 1a and Supplementary Table 4 ). 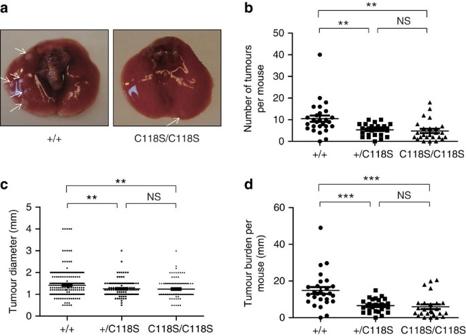Figure 4: Decreased urethane-induced lung tumorigenesis in mice with aKrasC118Sallele. (a) Visible lesions (arrows) of lungs from oneKras+/+(+/+) and oneKrasC118S/C118S(C118S/C118S) mouse 8 months after treatment with urethane. (b) Number of visible surface tumour lesions per mouse, (c) diameter of each visible surface tumour lesion and, (d) tumour burden, as defined by the sum of the diameters of all visible surface tumour lesions per mouse, fromKras+/+(+/+, 27 mice, 285 visible surface tumours),Kras+/C118S(+/C118S, 25 mice, 132 visible surface tumours) andKrasC118S/C118S(C118S/C118S, 25 mice, 121 visible surface tumours) mice 8 months after treatment with urethane. Bars: mean±s.e.m. NS: non-significant (P>0.05), **P<0.01 and ***P<0.001, as determined using one-way analysis of variance pluspost-hocBonferroni’s multiple comparison test. These mice were crossed with CMVCre transgenic mice to induce Cre-mediated recombination between the loxP sites flanking the Neo cassette. Successful excision of the Neo cassette was identified by PCR amplification of genomic DNA, yielding a 517-bp, instead of a 621-bp product, using primers P3 and P5, as well as by confirming the absence of the aforementioned 314 bp product using primers P3 and P4 ( Supplementary Fig. 1b ). The presence of CMVCre was identified by PCR amplification of genomic DNA using primers (P16 and P17, Supplementary Table 4 ) designed to generate a 100-bp PCR product unique to this transgene ( Supplementary Fig. 1b ). CMVCre;Kras +/C118S mice identified in this manner were then crossed with Kras +/+ mice to generate Kras +/C118S mice without CMVCre for use in subsequent experiments, again with the desired genotypes confirmed by similar PCR strategies. Finally, Kras +/C118S mice were crossed, generating Kras +/+ , Kras +/C118S and Kras C118S/C118S offspring, the genotype of which were identified by PCR amplification of genomic DNA using the aforementioned primer pair P3 and P5 ( Fig. 1a and Supplementary Table 4 ) that distinguished wild-type versus C118S Kras alleles by the amplification of a 621-bp versus a 517-bp product ( Fig. 1c and Supplementary Fig. 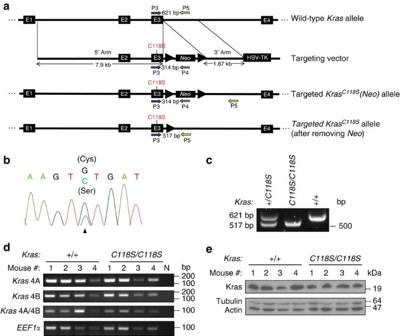6a ). Figure 1: Generation of mice with aKrasC118Sallele. (a) Schematic representation of homologous recombination (thin black lines) between the endogenous wild-typeKrasgene (E-numbered black boxes: exons, thick black lines: introns) and theKrasC118S-targeting vector (Neo:Neoselection marker; thick arrows:loxPrecombination sites; HSV-TK: HSV promoter-driven thymidine kinase-negative selection marker) as well as the resultant successfully targetedKrasC118Sknock-in allele before and after Cre-mediated recombination of the flankingloxPsites to excise theNeoselection marker. Coloured arrows: PCR primers used in genotyping. (b) Sequencing chromatogram of RT–PCR amplifiedKrasmRNA from a successfully targeted ES cell clone identifying the wild-type (G) and mutated (C) nucleotide at position 353 that changes the cysteine 118 to serine. (c) PCR amplification using the primer pair P3+P5 of genomic DNA from offspring of the indicated genotypes from crossingKras+/C118Smice. (d) RT–PCR amplification ofKrasmRNA from the lungs of fourKras+/+mice and fourKrasC118S/C118Smice (numbered 1, 2, 3 and 4) using primer pairs specific for the indicatedKrassplice variants (seeSupplementary Table 4). N: no DNA as a negative control reaction.EEF1α: loading control. (e) Immunoblot of lysates isolated from the lungs of fourKras+/+mice and fourKrasC118S/C118Smice (numbered 1, 2, 3 and 4) with an anti-Kras antibody. Tubulin and actin: loading controls. Figure 1: Generation of mice with a Kras C118S allele. ( a ) Schematic representation of homologous recombination (thin black lines) between the endogenous wild-type Kras gene (E-numbered black boxes: exons, thick black lines: introns) and the Kras C118S -targeting vector ( Neo : Neo selection marker; thick arrows: loxP recombination sites; HSV-TK: HSV promoter-driven thymidine kinase-negative selection marker) as well as the resultant successfully targeted Kras C118S knock-in allele before and after Cre-mediated recombination of the flanking loxP sites to excise the Neo selection marker. Coloured arrows: PCR primers used in genotyping. ( b ) Sequencing chromatogram of RT–PCR amplified Kras mRNA from a successfully targeted ES cell clone identifying the wild-type (G) and mutated (C) nucleotide at position 353 that changes the cysteine 118 to serine. ( c ) PCR amplification using the primer pair P3+P5 of genomic DNA from offspring of the indicated genotypes from crossing Kras +/C118S mice. ( d ) RT–PCR amplification of Kras mRNA from the lungs of four Kras +/+ mice and four Kras C118S/C118S mice (numbered 1, 2, 3 and 4) using primer pairs specific for the indicated Kras splice variants (see Supplementary Table 4 ). N: no DNA as a negative control reaction. EEF1α : loading control. ( e ) Immunoblot of lysates isolated from the lungs of four Kras +/+ mice and four Kras C118S/C118S mice (numbered 1, 2, 3 and 4) with an anti-Kras antibody. Tubulin and actin: loading controls. Full size image Characterization of the Kras C118S allele We confirmed that the strategy to introduce the G353>C transversion into the Kras gene did not overtly affect alternative splicing of terminal exons 4A and 4B, an important consideration as both splice forms are important for carcinogen-induced lung tumorigenesis [25] , [26] . Specifically, RT–PCR analysis with primers designed to amplify only Kras 4A or only Kras 4B detected both versions in lung tissue isolated from Kras +/+ and Kras C118S/C118S mice ( Fig. 1d and Supplementary Fig. 6b ). Similarly, we confirmed that this alteration of the Kras gene did not overtly affect protein expression, given that tumour initiation is sensitive to the level of Ras protein [21] . Specifically, immunoblot analysis revealed no detectable difference in the amount of Kras protein in lung tissue isolated from Kras +/+ versus Kras C118S/C118S mice ( Fig. 1e and Supplementary Figs 2 and 6c ). Finally, we demonstrate that introducing the C118S mutation into endogenous Kras gene can affect the ability of eNOS to stimulate the MAPK pathway. Specifically, mouse embryonic fibroblasts (MEFs) were isolated from two control Kras +/+ and two experimental Kras C118S/C118S embryos and immortalized with the SV40 early region. These four cell lines were then stably infected with a retrovirus encoding no transgene or the S1177D-activated mutant version of HA-tagged eNOS [27] , [28] . Lysates isolated seven independent times from the resultant eight cell lines were then immunoblotted for ectopic eNOS, endogenous Kras and tubulin, as well as total (T) and phosphorylated (P) Erk1/2. Although the normalized levels of P-Erk1/2 varied from experiment to experiment among the samples, on average there was a smaller fold increase in the normalized P-Erk1/2 levels upon expression of eNOS S1177D in Kras C118S/C118S compared with Kras +/+ MEFs (0.90±0.14 versus 3.21±0.91, P <0.02, Fig. 2 and Supplementary Fig. 6d ). 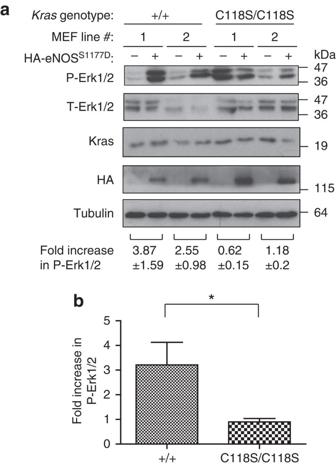Collectively, we conclude that the single G353>C transversion encoding the desired C118S mutation was successfully knocked into the Kra s locus with no overt effect on the expression of the resultant gene products. Figure 2: Reduced increase in P-Erk1/2 levels inKrasC118S/C118SMEFs upon expressing activated eNOS. (a) Immunoblot of HA-tagged ectopic eNOS, endogenous Kras and tubulin, as well as total (T) and phosphorylated (P) Erk1/2 from twoKras+/+and twoKrasC118S/C118SSV40-immortalized MEF cell lines in the absence or presence of HA-eNOSS1177D. Bottom: mean±s.e.m. of the indicated fold increase in P-Erk1/2 (normalized to T-Erk1/2) from immunoblot analysis of lysates derived seven independent times. (b) Mean±s.e.m. fold increase in P-Erk1/2 levels (normalized to T-Erk1/2) upon expression of eNOSS1177Dfrom lysates derived seven independent times from the twoKras+/+(+/+) or twoKrasC118S/C118S(C118S/C118S) SV40-immortalized MEF cell lines. *P<0.05, as determined by two-tailed unpaired Student’st-test. Figure 2: Reduced increase in P-Erk1/2 levels in Kras C118S/C118S MEFs upon expressing activated eNOS. ( a ) Immunoblot of HA-tagged ectopic eNOS, endogenous Kras and tubulin, as well as total (T) and phosphorylated (P) Erk1/2 from two Kras +/+ and two Kras C118S/C118S SV40-immortalized MEF cell lines in the absence or presence of HA-eNOS S1177D . Bottom: mean±s.e.m. of the indicated fold increase in P-Erk1/2 (normalized to T-Erk1/2) from immunoblot analysis of lysates derived seven independent times. ( b ) Mean±s.e.m. fold increase in P-Erk1/2 levels (normalized to T-Erk1/2) upon expression of eNOS S1177D from lysates derived seven independent times from the two Kras +/+ (+/+) or two Kras C118S/C118S (C118S/C118S) SV40-immortalized MEF cell lines. * P <0.05, as determined by two-tailed unpaired Student’s t -test. Full size image Kras C118S/C118S mice appear normal Identification of genotypes of 580 offspring from crossing Kras +/C118S mice revealed that there was no statistical difference between the observed frequency versus the expected Mendelian ratio of the three genotypes of Kras +/+ , Kras +/C118S and Kras C118S/C118S ( χ 2 test, P =0.545, Table 1 ). Kras C118S/C118S mice were also phenotypically indistinguishable from Kras +/+ mice ( Fig. 3a ). Weekly weight measurements, beginning at 8 weeks of age and continuing for another 17 weeks, revealed no statistical difference in the weight of either male or female mice between the Kras +/+ versus Kras C118S/C118S genotypes ( Fig. 3b,c ). The Kras −/− genotype is embryonic to neonatal lethal, and is characterized by defective cardiovascular function [29] . As heart defects are a hallmark of defective Kras function, we also compared the heart-to-body weight ratio between Kras +/+ versus Kras C118S/C118S mice, finding no significant difference between the two cohorts ( Fig. 3d ). Finally, Kras +/+ mice had a median lifespan of 847 days, whereas Kras C118S/C118S mice had a median lifespan of 670 days, but the difference was not significant ( Fig. 3e ). Collectively, these data indicate that mice with one or more Kras C118S alleles do not have any obvious developmental or physiological defects. 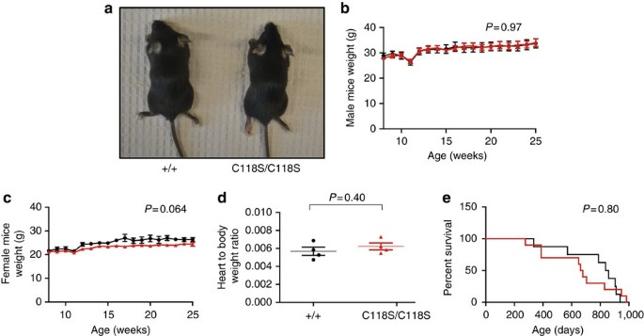Table 1 Expected and observed frequencies of offspring from crossing Kras +/C118S mice. Figure 3:KrasC118S/C118Smice have no overt phenotypes. (a) Photograph of aKras+/+(+/+) andKrasC118S/C118S(C118S/C118S) adult mouse at 3 weeks of age. (b,c) Mean body weight±s.e.m. of ([cirf ])Kras+/+versus (▴)KrasC118S/C118S(b) male (n=6 versus 5) and (c) female mice (n=4 versus 5) from 8 to 25 weeks of age. (d) Mean heart to body weight ratio±s.e.m. of 4-week-oldKras+/+(+/+) versusKrasC118S/C118S(C118S/C118S) mice (n=4). (e) Kaplan–Meier survival curves ofKras+/+(black line,n=8) versusKrasC118S/C118S(red line,n=10) mice.Pvalue was determined by multivariate analysis of variance test (b,c), two-tailed unpaired Student’st-test (d) and long-rank test (e). Full size table Figure 3: Kras C118S/C118S mice have no overt phenotypes. ( a ) Photograph of a Kras +/+ (+/+) and Kras C118S/C118S (C118S/C118S) adult mouse at 3 weeks of age. ( b , c ) Mean body weight±s.e.m. of ([cirf ]) Kras +/+ versus ( ▴ ) Kras C118S/C118S ( b ) male ( n =6 versus 5) and ( c ) female mice ( n =4 versus 5) from 8 to 25 weeks of age. ( d ) Mean heart to body weight ratio±s.e.m. of 4-week-old Kras +/+ (+/+) versus Kras C118S/C118S (C118S/C118S) mice ( n =4). ( e ) Kaplan–Meier survival curves of Kras +/+ (black line, n =8) versus Kras C118S/C118S (red line, n =10) mice. P value was determined by multivariate analysis of variance test ( b , c ), two-tailed unpaired Student’s t -test ( d ) and long-rank test ( e ). Full size image Reduced carcinogenesis in mice with a Kras C118S allele To determine the impact of the Kras C118S mutation on carcinogenesis, we assessed the effect of treating Kras +/+ , Kras +/C118S and Kras C118S/C118S mice with the carcinogen urethane (ethyl carbamate), which induces lung tumours characterized by oncogenic Q61R/L mutations in Kras [30] . We chose this approach to model a Kras mutation-positive cancer spontaneously arising from an environmental insult [30] in the lung, especially given the prevalence of KRAS mutations in human lung cancer [31] . As an important note, the Pas1 locus responsible for the different susceptibilities to urethane-induced tumorigenesis observed among inbred strains of mice maps to a region containing six genes, one being Kras [32] . Therefore, Kras +/C118S mice, which possess the Kras C118S allele from the 129S6/SvEvTac background, but the other native Kras allele from the C57/BL6 background (introduced during the excision of the Neo cassette), were crossed with Kras +/+ mice from the 129S6/SvEvTac background. Resultant Kras +/C118S mice were then crossed to generate Kras +/+ , Kras +/C118S and Kras C118S/C118S mice in which both Kras alleles originated from a 129S6/SvEvTac background. Cohorts of 27 Kras +/+ , 25 Kras +/C118S and 25 Kras C118S/C118S littermates from multiple breeding pairs were then intraperitoneally injected with urethane at 8 weeks of age. Eight months later, mice from all three cohorts were euthanized and lungs removed for analysis. Comparison of the number and size of visible surface lung lesions revealed that Kras +/C118S and Kras C118S/C118S mice developed fewer tumours with a smaller average tumour size, resulting in an overall reduction in tumour burden, as defined by the sum of the diameters of all visible surface tumours per mouse, compared with control Kras +/+ mice. There was no statistical difference in tumour number or size between the Kras +/C118S and Kras C118S/C118S cohorts ( Fig. 4a–d and Table 2 ). Binning tumours based on size, namely small (≤1 mm), medium (1–3 mm) or large (≥3 mm), revealed a significant shift ( χ 2 test, P =0.0014) from larger tumours in Kras +/+ mice to smaller tumours in Kras C118S/C118S mice ( Table 2 ). To independently validate these results, one lung from each of the mice in the three cohorts was formalin fixed, paraffin embedded, sectioned, haematoxylin and eosin (H&E)-stained, and the type and size of tumours analysed. Focusing on the most common type of lesion, adenomas were microscopically counted and binned as above as being small, medium or large. Again, there was a shift to smaller tumours in mice having one or more Kras C118S alleles. Specifically, large adenomas were only detected in Kras +/+ mice, and these mice also had a higher incidence of adenomas of medium size, whereas Kras +/C118S and Kras C118S/C118S mice had a statistically higher incidence of small-sized adenomas ( χ 2 test, P ≤0.01, Table 3 ). Collectively, these data demonstrate that the presence of the Kras C118S allele impairs urethane carcinogenesis. Figure 4: Decreased urethane-induced lung tumorigenesis in mice with a Kras C118S allele. ( a ) Visible lesions (arrows) of lungs from one Kras +/+ (+/+) and one Kras C118S/C118S (C118S/C118S) mouse 8 months after treatment with urethane. ( b ) Number of visible surface tumour lesions per mouse, ( c ) diameter of each visible surface tumour lesion and, ( d ) tumour burden, as defined by the sum of the diameters of all visible surface tumour lesions per mouse, from Kras +/+ (+/+, 27 mice, 285 visible surface tumours), Kras +/C118S (+/C118S, 25 mice, 132 visible surface tumours) and Kras C118S/C118S (C118S/C118S, 25 mice, 121 visible surface tumours) mice 8 months after treatment with urethane. Bars: mean±s.e.m. NS: non-significant ( P >0.05), ** P <0.01 and *** P <0.001, as determined using one-way analysis of variance plus post-hoc Bonferroni’s multiple comparison test. Full size image Table 2 Quantification of surface lung tumours from urethane-treated mice. Full size table Table 3 Histological quantification of lung adenomas from urethane-treated mice. Full size table To assess whether there was also an impact on tumour progression, lesions were graded [33] as being atypical adenomatous hyperplasia (AAH), adenoma (AD), or adenocarcinoma (AC) by histology ( Supplementary Fig. 3 ). This analysis revealed a similar tumour spectrum among the three genotypes. Specifically, regardless of the genotype, the majority of the tumours were AD, with only a few AAH and an infrequent number of AC in each group ( Supplementary Table 1 ). AD lesions were further classified [34] into papillary, solid or mixed solid/papillary subtypes ( Supplementary Fig. 3 ). There was no significant difference in the incidence of solid AD among the three groups, although the Kras +/C118S mice appeared to have fewer papillary AD and more mixed solid/papillary AD ( Supplementary Table 2 ). Finally, immunohistochemical analysis of lung lesions in four to six random microscope fields from five mice each having the genotypes Kras +/+ , Kras +/C118S or Kras C118S/C118S after treatment with urethane did not show any overt difference in the level of Ras signalling, as assessed by P-Erk1/2 or P-Akt immunostaining, or in proliferation, as assessed by Ki67 immunostaining, with the exception of reduced P-Akt in the Kras +/C118S cohort ( Supplementary Fig. 4a,b ). Collectively, these data point towards a negative effect of the Kras C118S allele, particularly at the stage of tumour initiation. Similar tumorigenesis between Kras LSL-G12D/+ and Kras LSL-G12D/C118S mice In the urethane-induced lung tumour model, typically only one Kra s allele acquires an oncogenic mutation. Although the oncogenic Kras allele is well established to promote tumorigenesis, the remaining non-oncogenic allele has actually been found to be tumour suppressive in some settings [35] . As such, the observed negative effect of the Kras C118S allele on lung tumourigenesis is ostensibly due to the C118S mutation either suppressing the tumorigenic activity of oncogenic Kras allele and/or enhancing tumour suppressive effect of the remaining non-oncogenic Kras allele. To test the latter possibility, we took advantage of mice with a conditionally oncogenic LSL-Kras G12D allele to compare the effect of the remaining Kras allele with or without a C118S mutation on lung tumorigenesis. In more detail, infection of lung tissue upon intranasal administration of adenovirus encoding Cre (AdCre) induces recombination of loxP sites flanking a transcriptional/translational STOP sequence ( LSL ) upstream of Kras harbouring a G12D oncogenic mutation, thereby permitting expression of the Kras G12D allele, which promotes lung tumorigenesis [36] . Thus, LSL-Kras G12D/+ mice were crossed with Kras +/C118S mice in which both Kras alleles were of the 129S6/SvEvTac background. Cohorts of 21 resultant Kras LSL-G12D /+ and 17 Kras LSL-G12D/C118S littermates from multiple breeding pairs were treated intranasally with AdCre at 8 weeks of age. Four months later mice from both cohorts were euthanized and lungs removed for analysis. Quantification of the number, size and total burden of visible surface lesions revealed no statistical difference between the two cohorts ( Fig. 5a–c ). The sizes of these cohorts are powered to detect differences in the number, burden and size of 1.52, 1.78 and 0.52 mm, respectively. Similarly, microscopic quantification of the number of lesions in H&E-stained lung sections from these mice ( Supplementary Fig. 5 ) revealed no significant difference between these two cohorts ( Fig. 5d ). Thus, the Kras C118S allele does not appear to confer any overt change to the tumour-suppressive activity to the non-oncogenic allele in a lung tumour model driven by Kras G12D . 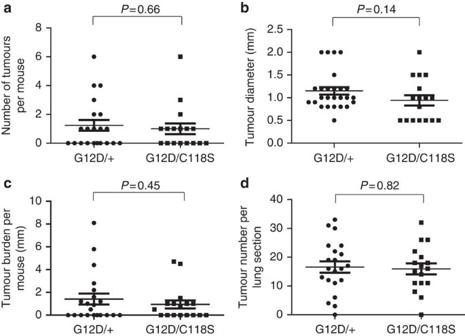Figure 5:KrasG12D-driven lung tumorigenesis is similar when the remainingKrasallele is wild-type or C118S. (a) Number of visible surface tumour lesions per mouse, (b) diameter of each visible surface tumour lesion, (c) tumour burden, as defined by the sum of the diameters of all visible surface tumour lesions per mouse, and (d) number of lesions detected in each H&E-stained section fromKrasLSL-G12D/+(G12D/+, 21 mice, 26 visible surface tumours) versusKrasLSL-G12D/C118S(G12D/C118S, 17 mice, 17 visible surface tumours) mice 4 months after intranasal administration of AdCre. Bars: mean±s.e.m.Pvalues were determined using two-tailed unpaired Student’st-test. Figure 5: Kras G12D -driven lung tumorigenesis is similar when the remaining Kras allele is wild-type or C118S. ( a ) Number of visible surface tumour lesions per mouse, ( b ) diameter of each visible surface tumour lesion, ( c ) tumour burden, as defined by the sum of the diameters of all visible surface tumour lesions per mouse, and ( d ) number of lesions detected in each H&E-stained section from Kras LSL-G12D/+ (G12D/+, 21 mice, 26 visible surface tumours) versus Kras LSL-G12D/C118S (G12D/C118S, 17 mice, 17 visible surface tumours) mice 4 months after intranasal administration of AdCre. Bars: mean±s.e.m. P values were determined using two-tailed unpaired Student’s t -test. Full size image Mutational bias against the Kras C118S allele We next tested whether there was a bias of oncogenic mutations induced by urethane in either the native or C118S Kras allele in Kras +/C118S mice. To this end, RNA was extracted from 65 lung tumours from 20 Kras +/C118S mice treated with urethane. Kras mRNA was then RT–PCR amplified, cloned and sequenced to identify the allelic origin (native or C118S) and mutation status (wild-type or oncogenic). No oncogenic mutation was detected in either Kras allele in 21 tumours, only one allele was recovered in another 9 tumours and a mutation was detected in both alleles in 3 tumours. As such, these samples were excluded from the analysis. Of the remaining 32 tumours (derived from 15 Kras C118S/+ mice) in which both Kras alleles were recovered and there was an oncogenic mutation in only one of the alleles, 20 tumours had an oncogenic Q61R/L mutation in the native Kras allele, whereas 12 had the mutation in the Kras C118S allele ( Fig. 6 and Supplementary Table 3 ). This almost twofold enrichment in mutations recovered in the native Kras allele was significantly different from the expected frequency, assuming the incidence of oncogenic Q61R/L mutations occurring on the native Kras and the Kras C118S allele was both 50% ( χ 2 test, P =0.0455). 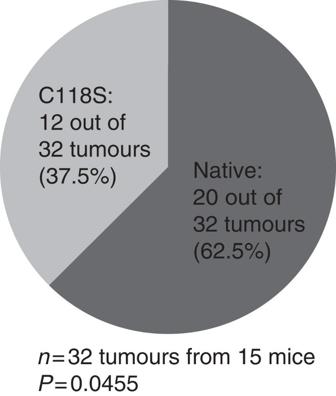Figure 6: Oncogenic Q61 mutations occur preferentially on the nativeKrasallele. Pie chart of the number and percent of Q61R/L oncogenic mutations found in the native versus the C118SKrasallele, as determined by RT–PCR amplification and sequencing ofKrasmRNA isolated from 32 lung lesions from 15Kras+/C118Smice 8 months after treatment with urethane.Pvalue was determined using theχ2test to compare the difference between the observed and the expected frequency. Figure 6: Oncogenic Q61 mutations occur preferentially on the native Kras allele. Pie chart of the number and percent of Q61R/L oncogenic mutations found in the native versus the C118S Kras allele, as determined by RT–PCR amplification and sequencing of Kras mRNA isolated from 32 lung lesions from 15 Kras +/C118S mice 8 months after treatment with urethane. P value was determined using the χ 2 test to compare the difference between the observed and the expected frequency. Full size image The above results suggest a bias against oncogenic mutations in the Kras C118S allele. Although preliminary experiments revealed that ectopic Kras Q61L,C118S and Kras Q61L behaved rather similarly with regards to signalling, transformation and oncogene-induced growth arrest, there did appear to be a potential consequence of mutating C118 in the G13D oncogenic mutant background. Specifically, Kras C118S/C118S MEFs immortalized with the SV40 early region and transformed with either Kras G13D,C118S or Kras G13D were treated with epidermal growth factor (EGF) to stimulate GEF activity, given the potential involvement of GEFs in activating oncogenic Ras proteins [37] , [38] . Lysates derived three independent times from these two cell lines were then immunoblotted to detect ectopic Kras, endogenous tubulin, as well as total (T) and phosphorylated (P) Erk1/2. On average, this analysis revealed a trend towards a lower normalized P-Erk1/2 level upon EGF treatment in the Kras G13D,C118S compared with Kras G13D -transformed MEFs ( Fig. 7a,b and Supplementary Fig. 6e ). To exclude an involvement of wild-type Hras and Nras isoforms [20] , [39] , the Kras C118S/C118S genotype was crossed into an Hras −/− ;Nras −/− background to generate Kras C118S/C118S ;Hras −/− ;Nras −/− MEFs, which were then immortalized with the SV40 early region and transformed with either Kras G13D,C118S or Kras G13D . Based on three independent experiments, on average there was a decrease in the normalized P-Erk1/2 levels upon EGF treatment in the Kras G13D,C118S compared with the Kras G13D -transformed Kras C118S/C118S ;Hras −/− ;Nras −/− MEFs ( Fig. 7c,d and Supplementary Fig. 6f ). 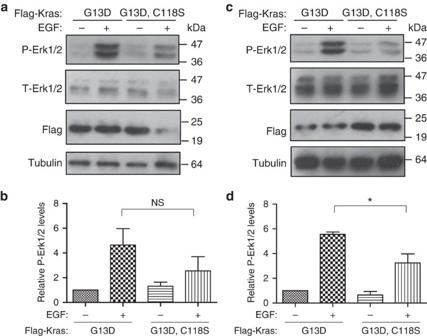Figure 7: Reduced increase in P-Erk1/2 levels in MEFs transformed with KrasG13D,C118Supon EGF treatment. Immunoblot of Flag-tagged ectopic Kras, tubulin, as well as total (T) and phosphorylated (P) Erk1/2 from (a)KrasC118S/C118Sor (c)Nras−/−;Hras−/−;KrasC118S/C118SMEFs immortalized with the SV40 early region and transformed with either Flag-KrasG13Dor Flag-KrasG13D,C118Sin the absence or presence of EGF stimulation. (b,d) Mean±s.e.m. of P-Erk1/2 levels (normalized to T-Erk1/2) from three independent experiments using lysates from (b)KrasC118S/C118Sor (d)Nras−/−;Hras−/−;KrasC118S/C118SMEFs immortalized with the SV40 early region and transformed with either Flag-KrasG13Dor Flag-KrasG13D,C118Sin the absence or presence of EGF stimulation. NS: non-significant (P>0.05). *P<0.05, as determined using one-way analysis of variance pluspost-hocBonferroni’s multiple comparison test. Figure 7: Reduced increase in P-Erk1/2 levels in MEFs transformed with Kras G13D,C118S upon EGF treatment. Immunoblot of Flag-tagged ectopic Kras, tubulin, as well as total (T) and phosphorylated (P) Erk1/2 from ( a ) Kras C118S/C118S or ( c ) Nras −/− ;Hras −/− ;Kras C118S/C118S MEFs immortalized with the SV40 early region and transformed with either Flag-Kras G13D or Flag-Kras G13D,C118S in the absence or presence of EGF stimulation. ( b , d ) Mean±s.e.m. of P-Erk1/2 levels (normalized to T-Erk1/2) from three independent experiments using lysates from ( b ) Kras C118S/C118S or ( d ) Nras −/− ;Hras −/− ;Kras C118S/C118S MEFs immortalized with the SV40 early region and transformed with either Flag-Kras G13D or Flag-Kras G13D,C118S in the absence or presence of EGF stimulation. NS: non-significant ( P >0.05). * P <0.05, as determined using one-way analysis of variance plus post-hoc Bonferroni’s multiple comparison test. Full size image We report that mutating C118 of endogenous Kras to serine suppressed urethane-induced lung tumorigenesis. We recognize that it is formally possible that the recombined loxP sites introduced into the intron during the generation of the Kras C118S allele could underlie this effect rather than the C118S mutation. However, such a possibility seems less likely given that the Kras C118S allele yielded both Kras 4A and Kras 4B transcripts, produced similar levels of protein compared with the native Kras allele, and had no observable phenotype in a homozygous setting. The C118S mutation also inhibits the ability of Ras proteins to be activated in the presence of reactive nitrogen or oxygen species [6] , [8] , [10] , [12] , [17] , [18] , [22] , [23] , [24] . Thus, prior research additionally supports a plausible correlation between the mutation of the redox-reactive moiety at the C118 site and the observed reduction in tumorigenicity in mice with one or two Kras C118S alleles. Introducing the C118S mutation into the remaining Kras allele in the LSL-Kras G12D model of lung cancer had no obvious effect on the number or size of resultant tumours, suggesting that the C118S mutation does not confer any overt change to the tumour-suppressive activity of the non-oncogenic allele. This does not, however, exclude a role for the C118 in the wild-type Kras protein in other settings. Indeed, the C118S mutation in wild-type Hras and Nras inhibits the xenograft tumour growth of some cancer cell lines [20] . As such, the effect of mutating this residue may be temporal or context-dependent in cancer, consistent with the highly variable effects of, for example, nitric oxide on tumorigenesis [40] . Nevertheless, extrapolating the results from this experiment, we suggest that the reduction of lung tumours in urethane-treated Kras C118S/+ or Kras C118S/C118S mice may be more related to the oncogenic, rather than remaining non-oncogenic Kras allele. Sequencing analysis suggests a preference of oncogenic mutations in the native compared with the C118S allele in tumours from Kras +/C118S mice treated with urethane. It is formally possible that carcinogens cause fewer mutations in the Kras C118S allele by some unknown mechanism. However, the C118S is only a point mutation, lies more than 2 kb away and in a completely different exon from where the Q61 oncogenic mutations occur, and is well established to block redox-dependent activation of Ras [6] , [8] , [10] , [12] , [17] , [18] , [22] , [23] , [24] . Thus, we favour a model whereby an oncogenic mutation in the Kras C118S allele is less likely to lead to productive tumorigenesis. Accumulating evidence suggests a potential role of GEFs in activating oncogenic Ras proteins [37] , [38] , and in this regard, there was a difference in the ability of EGF to stimulate the MAPK pathway in cells transformed by Kras G13D,C118S versus Kras G13D . However, the relationship of NO and urethane tumorigenesis is undoubtedly more complex. NO can be generated from urethane derivatives in the appropriate conditions in vitro [41] and iNOS knockout mice are resistant to this carcinogen [42] . As such, the apparent preference of oncogenic mutations in the native compared with the C118S allele of Kras awaits a biochemical or cellular explanation. In summary, these results indicate that urethane carcinogenesis is reduced in mice with the Kras C118S allele, an effect that may be linked to the oncogenic rather than the native Kras version of the gene. Plasmids pBabeNeo-SV40-T/t-Ag (encoding the early region of SV40) was described previously [20] , [43] . pBabeBleo-eNOS S1177D -HA was generated by introducing a mutation resulting in a S1177D amino-acid change into C-terminal HA-epitope-tagged eNOS cDNA [20] . pBabePuroFlag-Kras G13D was generated by introducing a mutation resulting in a G13D amino-acid change into N-terminal FLAG-epitope-tagged human Kras cDNA [20] . pBabePuroFlag-Kras G13D,C118S was generated by introducing a mutation resulting in a C118S amino-acid change into the aforementioned pBabePuroFlag-Kras G13D plasmid. Animals All animal experiments were approved by an Institutional Animal Care and Use Committee at Duke University. 129S6/SvEvTac mice were from Taconic. C57BL/6 mice (C57BL/6NJ), CMVCre transgenic mice (B6.C-Tg (CMV-cre)1Cgn/J) and Kras LSL-G12D transgenic mice (129S/Sv- Kras tm4Tyj /J) were obtained from Jackson Laboratory. Kras C118S knock-in mice were generated at Transgenic Mouse Facility of Duke Cancer Institute. The described targeting vector ( Fig. 1a ) was linearized with Not I and electroporated into W4 ES cells from 129S6/SvEvTac mice, followed by positive selection with G418 and negative selection with ganciclovir. RNA was isolated from individual ES cell clones, and RT–PCR was performed with primers P1 and P2 to amplify Kras cDNA ( Supplementary Table 4 ). PCR products were resolved in 2% agarose gels, purified by a gel purification kit (Qiagen), and sequenced to confirm the Kras C118S mutation. One successfully targeted clone was injected into C57BL/6 blastocysts, which were then implanted into pseudo-pregnant females to generate chimeras. Male chimeras were bred with female C57BL/6 mice, and offspring with germline transmission of the Kras C118S(Neo) allele were identified by PCR of genomic DNA with primer pairs P3+P4 specific for the Kras C118S allele and P3+P5 specific for the wild-type allele ( Supplementary Table 4 ) as well as direct sequencing of Kras RT–PCR products from lung tissue. Male Kras +/C118S(Neo) mice were bred with female CMVCre transgenic mice to excise the Neo cassette. The genotypes of offspring were identified by PCR of genomic DNA using the primer pair P3+P5 to identify the wild-type Kras allele and the Kras C118S allele lacking the Neo cassette. Absence of the Neo cassette was also confirmed with primer pair P3+P4, which does not generate a product when the Neo cassette is deleted. CMVCre;Kras +/C118S mice were then crossed with Kras +/+ mice to generate Kras +/C118S mice without CMVCre for use in all the animal studies. Kras +/C118S mice were crossed to generate Kras +/+ , Kras +/C118S and Kras C118S/C118S mice, whose genotypes were again identified by PCR of genomic DNA using the primer pair P3+P5. Kras +/C118S mice were further crossed into Nras −/− ; Hras −/− background to generate Nras −/− ; Hras −/− ; Kras +/C118S mice. Generation of MEFs and cell culture All the cells were maintained in Dulbecco’s modified Eagle’s medium (DMEM) supplemented with 10% fetal bovine serum (FBS) and incubated at 37 °C in a 5% CO 2 incubator. Kras +/+ and Kras C118S/C118S MEFs were prepared from embryos from Kras C118S/+ females bred with a Kras C118S/+ male. Embryos (E13-E16) were dissected from euthanized pregnant Kras C118S/+ females and washed with sterile PBS. The head of each embryo was removed for isolation of genomic DNA and identification of genotypes by PCR using primers P3+P5 as described above. The remaining embryos were cut into pieces in a sterile dish and incubated with 1 ml 0.25% trypsin at 37 °C in a 5% CO 2 incubator for 30–45 min. The trypsinized cells were then mixed with 10 ml 10% FBS DMEM and incubated at 37 °C in a 5% CO 2 incubator for further experiments. Nras −/− ; Hras −/− ; Kras C118S/C118S MEFs were prepared as above from embryos from an Nras −/− ; Hras −/− ; Kras C118S/+ female bred with an Nras −/− ; Hras −/− ; Kras C118S/+ male. Primary MEF lines were immortalized by stable infection [43] with retroviruses derived from pBabeNeo-SV40-T/t-Ag. In some cases these cells were further stably infected [43] with retroviruses derived from pBabeBleo, pBabeBleo-eNOS S1177D -HA, pBabePuroFlag-Kras G13D or pBabePuroFlag-Kras G13D,C118S . Where indicated, immortalized MEFs were serum starved by incubating with 0.5% FBS DMEM overnight and harvested the next day. Where indicated, immortalized MEFs were also treated with 100 ng μl −1 EGF (Sigma) for 5 min at 37 °C in a 5% CO 2 incubator before being harvested on ice. Immunoblot analysis Cells or lung tissue were lysed with RIPA buffer (1% NP-40, 20 mM Tris, pH 8.0, 137 mM NaCl, 10% glycerol, 2mM EDTA) and protein concentrations quantified by Bradford assay (Bio-Rad). Equal amounts of protein lysates (50 μg) were resolved by SDS–polyacrylamide gel electrophoresis, transferred to a polyvinylidene difluoride membrane and immunoblotted with primary antibodies: anti-Kras F234 (Santa Cruz, sc-30, diluted 1:200), anti-Flag M2 (Sigma, F1804, diluted 1:500), anti-HA (Covance, diluted 1:1,000), anti-β-actin (Sigma, A2228, diluted 1:10,000), anti-β-tubulin (Sigma, T5201, diluted 1:2,000), anti-Erk1/2 (Santa Cruz, sc-94, diluted 1:2,000) or anti-P (Thr 202/Tyr 204)-Erk1/2 (Santa Cruz, sc-7383, diluted 1:500), followed by incubation with either goat anti-rabbit (Santa Cruz, sc-2004, diluted 1:5,000) or anti-mouse (Invitrogen, G21040, diluted 1:10,000) IgG-HRP-conjugated secondary antibodies and detected by ECL (GE Healthcare). Bands of targeted protein in scanned images were quantified using Image J software and normalized. RT–PCR RNA was extracted from ES cells, lung tissue or lung tumours with the RNA-BEE reagent according to the manufacture’s protocol (Fisher Scientific). 0.5–2 μg of RNA was reverse transcribed using Omniscript RT kit (Qiagen) and Oligo dT (Qiagen) as primers. Resultant cDNA was used as a template to amplify targets of interest using the primers listed in Supplementary Table 4 . Urethane carcinogenesis Kras +/C118S mice (without CMVCre) were bred with Kras +/+ mice in 129S6/SvEvTac background. Resultant Kras +/C118S mice were then crossed to generate Kras +/+ , Kras +/C118S and Kras C118S/C118S littermates in which both Kras alleles originated from a 129S6/SvEvTac background. Twenty-five to twenty-seven male and female mice of each genotype were ultimately compared with detect a measurable difference in tumour parameters between control and experimental cohorts. A total of 38 male and 39 female mice at 2 months of age were intraperitoneally injected with urethane (1 mg g −1 body weight) [35] . Weight and behaviour were monitored twice weekly starting at 3 months post injection. Eight months after injection, mice were euthanized, and lungs were inflated with PBS and harvested for analysis. Lung surface tumours were counted under a dissecting microscope. Tumour diameter was determined using micro-calipers. Mice that reached moribundity end points before 8 months were excluded from the final analysis. The investigator was blinded to the genotype when injecting urethane as well as when assessing tumour number and size. Ad-Cre-induced lung tumorigenesis Kras +/C118S mice in which both Kras alleles originated from a 129S6/SvEvTac background were bred with LSL-Kras G12D/+ mice to generate Kras LSL-G12D/+ and Kras LSL-G12D/C118S mice. Seventeen to twenty-one male and female mice of each genotype were ultimately compared to detect a measurable difference in tumour parameters between control and experimental cohorts. Nine male and twenty-nine female mice were infected with 6 × 10E 6 p.f.u. of AdCre virus at 2 months of age [36] . Weight and behaviour were monitored twice weekly starting at 3 months post-AdCre. Four months after AdCre administration, mice were euthanized and lungs were inflated with PBS and harvested for analysis. Surface tumours were counted under a dissecting microscope. Tumour diameter was determined using micro-calipers. Mice that reached moribundity end points before 4 months were excluded from the final analysis. The investigator was blinded to the genotype when administrating AdCre as well as when assessing tumour number and size. Histological analysis Left lobes of lungs from the indicated mice (see above) were fixed in 10% neutral buffered formalin overnight, dehydrated in 70% ethanol and paraffin embedded. 5 μm-thick sections were cut from each sample, mounted on glass slides and stained with H&E. A total of 77 lung sections were reviewed by two pathologists (D.M.C. and J.C.) who were masked to the study design and blinded to the genotype. The number and type (AAH, AD and/or AC) of lesions were quantified in each sample. Adenomas were further classified by size (≤1, 1–3 or ≥3 mm) and histological subtype (solid, papillary or mixed solid-papillary) [34] . Immunohistochemistry Left lobes of lungs from the indicated mice (see above) were fixed in 10% neutral buffered formalin overnight, dehydrated in 70% ethanol and paraffin embedded. 5 μm-thick sections were cut from each sample, mounted on glass slides and subjected to epitope retrieval and stained with anti-P(Thr 202/Tyr 204)-Erk1/2 (Cell Signaling, 4376), anti-P(Ser473)-Akt (Cell Signaling, 4060) or anti-Ki67 (Thermo Scientific, RM9106) antibodies followed by peroxidase-based detection with Vectastain Elite ABC Kits (Vector Labs) and counterstained with haematoxylin. Photographs were taken of four to six high-power (× 20) random fields with tumour areas on an Olympus Vanox S microscope (Olympus). Images were blinded and tumours were circumscribed in stained tissue images with the freehand selection tool in Image J, and the total area of the tumour in pixels was recorded. Tumour images were copied and pasted to new, blank images and colour threshold was applied to determine positive-staining areas, using the same parameters for each tumour image. Areas staining positive by these parameters were selected and the positive staining area in pixels was recorded. The percentage of positive-staining area was calculated by dividing the positive-staining area of the tumour in pixels by the total area of tumours in pixels. Kras mutation analysis Lung tumours arising in urethane-treated Kras +/C118S mice (see above) were removed with the aid of a dissection microscope. A measure of 500 ng of RNA isolated from the tumours were RT–PCR amplified (see above) using the primer pair P6+P7 containing Hin dIII and Sac I sites, respectively ( Supplementary Table 4 ). Resultant products were cloned into the Hin dIII and Sac I sites of pBluescript vector (from Addgene), after which 12 positive clones from each ligation reaction were sequenced using T7 promoter (Eton Bioscience) to determine whether the clone corresponded to the native or C118S allele of Kras , and whether the clone had an oncogenic mutation (at position G12, G13 and Q61). Statistical analysis Data were presented as mean values±standard error of the mean (s.e.m.). Most statistical analyses were performed with Graphpad Prism 5 software. The two-tailed unpaired Student’s t -test was used to compare two groups. The one-way analysis of variance plus post-hoc Bonferroni’s multiple comparison tests were used to compare three or more groups. The multivariate analysis of variance test was used to compare mice weight change over time between two groups, whereas the long-rank test was performed to compare the survival between two groups. The χ 2 test was used to analyse difference in frequency (between the observed versus the expected or between two groups) based on contingency tables. P values <0.05 were considered significant. How to cite this article : Huang, L. et al . Decreased tumorigenesis in mice with a Kras point mutation at C118. Nat. Commun. 5:5410 doi: 10.1038/ncomms6410 (2014).